A designer cell-based histamine-specific human allergy profiler Allergic disorders are markedly increasing in industrialized countries. The identification of compounds that trigger the immunoglobulin E-dependent allergic reaction remains the key to limit patients’ exposure to critical allergens and improve their quality of life. Here we use synthetic biology principles to design a mammalian cell-based allergy profiler that scores the allergen-triggered release of histamine from whole-blood-derived human basophils. A synthetic signalling cascade engineered within the allergy profiler rewires histamine input to the production of reporter protein, thereby integrating histamine levels in whole-blood samples with remarkable sensitivity and a wide dynamic range, allowing for rapid results or long-term storage of output, respectively. This approach provides non-intrusive allergy profiles for the personalized medicine era. Synthetic biology, the emerging life science that uses engineering principles to assemble standardized biological parts in a systematic, rational and predictable manner to program novel cellular behaviour [1] , [2] , has significantly advanced the design of synthetic gene networks and signalling cascades that provide new treatment strategies for high-prevalence medical conditions [3] , [4] . For example, designer circuits are leading the way for next-generation anti-infectives [5] , [6] , cancer kill switches are being used to monitor, score and eliminate neoplastic cells [7] , [8] and prosthetic networks have been successfully validated for the treatment of metabolic disorders, such as gouty arthritis [9] and obesity [10] in animal models. With the advent of personalized medicine, diagnostic technologies are currently being revisited as a central strategy to discover, prevent and improve treatment of a variety of medical conditions. Allergies, such as hay fever, food allergies, eczema or allergic asthma, represent a major health burden in industrialized countries. Excessive activation of mast cells and basophil granulocytes upon exposure to allergen-bound immunoglobulin E (IgE) results in intracellular Ca 2+ -dependent signal transduction that triggers the release of vast levels of histamine from their granules. Histamine mediates allergic symptoms by binding and activating a family of G protein-coupled receptors, histamine receptors H1–4 (HRH1–4), which are differentially expressed by cells of various tissues, including immune, smooth muscle and endothelial cells [11] . Because the responsible allergy trigger often remains elusive, diagnostic allergy tests based on diverse in vivo and in vitro methods are crucial to prevent allergen exposure and to design specific therapeutic interventions [12] . The frequently used skin prick test is reproducible when performed by trained health professionals but requires direct contact between the allergen and the patient, which results in discomfort and the potential risk of anaphylaxis in certain patient groups [13] , [14] . In contrast, the in vitro quantification of specific, free IgE antibodies in human blood allows for the simultaneous screening of a multitude of allergens; however, the presence of IgE antibodies does not necessarily correlate with clinical symptoms [12] , [15] . Also, much effort has been made to mimic the allergic reaction in a test tube using whole blood followed by measurement of allergen-induced effector cell activation by quantification of specific surface-displayed proteins or mediator release [16] , [17] . For example, the basophil activation test utilizes cell-surface expression of CD63 as a marker for basophil activation quantified by flow cytometry [18] . The histamine release test simulates mediator release including histamine, which can be subsequently detected in the serum [15] , [19] . Current histamine-quantification assays include chromatography, fluorescence and immunoassay methods, which require large sample volumes and show a narrow dynamic range [17] . Also, to reach the high level of sensitivity needed for diagnostic purposes, most histamine-quantification technologies require partial enrichment of leukocytes or chemical derivatization of histamine, which involves time-consuming, multi-step sample preparations and sophisticated equipment [20] , [21] . Here, we report on a synthetic biology-inspired designer cell-based approach for the precise profiling of allergies in human whole-blood samples. Exposure of human blood to an array of allergens triggers an allergen-specific release of histamine by immune effector cells, such as basophil granulocytes circulating in the donor’s blood, thereby replicating the patient-specific allergic reaction in the body. The histamine levels are precisely scored by mammalian designer cells engineered with a synthetic signalling cascade rewiring histamine input to production of reporter proteins. This cell-based allergy profiler pioneers the use of synthetic biology principles for next-generation diagnostics. The histamine sensor device (HSD) consists of a synthetic histamine-responsive signalling cascade in which the G protein-coupled receptor HRH2 senses extracellular histamine levels ( Fig. 1a ) and triggers G s -protein-mediated activation of adenylate cyclase, which in turn converts ATP to cyclic AMP (cAMP). This second messenger molecule binds regulatory subunits of protein kinase A, whose catalytic subunits translocate into the nucleus where they phosphorylate the cAMP-responsive binding protein 1, which binds and activates synthetic P CRE promoters driving reporter gene expression ( Fig. 1a ). Rewiring of HRH2 to reporter gene expression provides a precise quantitative readout for extracellular histamine levels encountered by the designer cells. As a first step, we screened for best-performing components, including different potential target promoters ( Supplementary Fig. 1a ), various HRH2-driving constitutive promoters ( Supplementary Fig. 1b ) and a set of parental cell lines ( Supplementary Fig. 1c ). Experiments involving the co-transfection of the constitutive HRH2 expression vector pCK120 (P hEF1α - HRH2 -pA) with a P CRE -driven SEAP (secreted alkaline phosphatase) expression construct pCK53 (P CRE - SEAP -pA) into HEK-293 cells showed the best overall performance ( Supplementary Fig. 1a–c ). pCK120/pCK53-co-transfected HEK-293 cells (HSD SEAP ) were highly sensitive to histamine and dose dependently controlled reporter gene expression over a wide histamine concentration range (1–100 nM), covering even the lower physiological histamine levels in the human blood ( Supplementary Fig. 1d ) [22] . The high histamine sensitivity of the HSD was also confirmed by real-time monitoring of the histamine-responsive production of the intracellular fluorescent reporter gene Citrine (pDA134, P CRE - Citrine -pA) in pCK120/pDA134-co-transfected HEK-293 cell populations (HSD Citrine ) ( Fig. 1b ). 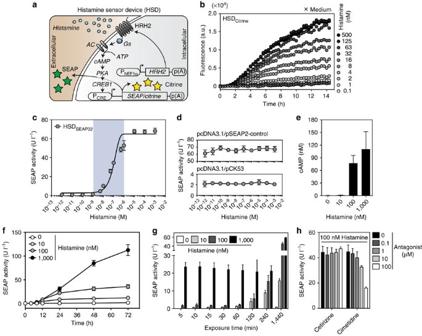Figure 1: Characterization of the histamine-triggered transgene switch. (a) Illustration of the histamine sensor device (HSD). Following constitutive expression by the human elongation factor 1 alpha promoter (PhEF1α), the histamine receptor H2 (HRH2) localizes to the plasma membrane. The G protein-coupled receptor HRH2 senses extracellular histamine and triggers Gs-mediated activation of adenylate cyclase (AC), which converts ATP to cyclic AMP (cAMP). cAMP binds the regulatory subunits of protein kinase A (PKA), whose catalytic subunits translocate into the nucleus where they phosphorylate the cAMP-responsive binding protein 1 (CREB1). Subsequently, CREB1 binds and activates a synthetic promoter (PCRE), which drives the expression of intracellular (Citrine) or secreted (SEAP) reporter proteins. (b) Real-time monitoring of histamine-triggered cellular fluorescence of HSDCitrine-engineered cell populations in a microplate reader. The plot shows the mean of three experiments. (c) Histamine sensitivity of transgenic HSDSEAP32cells. The data points were fitted using a sigmoidal dose-response curve. The blue translucent background represents the physiological range of histamine concentrations found in human blood. (d) Effect of histamine on the SEAP expression of HEK-293 cells with pcDNA3.1 and either pSEAP2-control (PSV40-SEAP-pA) or pCK53 (PCRE-SEAP-pA). (e) Profiling of the histamine-dependent intracellular cAMP surge in HSDSEAP32cells. (f) SEAP expression kinetics of HSDSEAP32cells exposed to different physiological histamine concentrations. (g) Impact of different histamine doses and induction time on HSDSEAP32-mediated SEAP expression. (h) Influence of specific HRH1 (cetirizine) and HRH2 (cimetidine) antagonists on HSDSEAP32-mediated SEAP expression. The data represent the means±s.d. (n≥3 experiments). Figure 1: Characterization of the histamine-triggered transgene switch. ( a ) Illustration of the histamine sensor device (HSD). Following constitutive expression by the human elongation factor 1 alpha promoter (P hEF1α ), the histamine receptor H2 (HRH2) localizes to the plasma membrane. The G protein-coupled receptor HRH2 senses extracellular histamine and triggers G s -mediated activation of adenylate cyclase (AC), which converts ATP to cyclic AMP (cAMP). cAMP binds the regulatory subunits of protein kinase A (PKA), whose catalytic subunits translocate into the nucleus where they phosphorylate the cAMP-responsive binding protein 1 (CREB1). Subsequently, CREB1 binds and activates a synthetic promoter (P CRE ), which drives the expression of intracellular (Citrine) or secreted (SEAP) reporter proteins. ( b ) Real-time monitoring of histamine-triggered cellular fluorescence of HSD Citrine -engineered cell populations in a microplate reader. The plot shows the mean of three experiments. ( c ) Histamine sensitivity of transgenic HSD SEAP32 cells. The data points were fitted using a sigmoidal dose-response curve. The blue translucent background represents the physiological range of histamine concentrations found in human blood. ( d ) Effect of histamine on the SEAP expression of HEK-293 cells with pcDNA3.1 and either pSEAP2-control (P SV40 - SEAP -pA) or pCK53 (P CRE - SEAP -pA). ( e ) Profiling of the histamine-dependent intracellular cAMP surge in HSD SEAP32 cells. ( f ) SEAP expression kinetics of HSD SEAP32 cells exposed to different physiological histamine concentrations. ( g ) Impact of different histamine doses and induction time on HSD SEAP32 -mediated SEAP expression. ( h ) Influence of specific HRH1 (cetirizine) and HRH2 (cimetidine) antagonists on HSD SEAP32 -mediated SEAP expression. The data represent the means±s.d. ( n ≥3 experiments). Full size image To evaluate whether the stable chromosomal integration of the HSD components into HEK-293 cells would further improve sensitivity and switching performance, we selected stable HSD SEAP (poly)clonal cell populations and profiled reporter gene expression after induction with 100 nM histamine ( Supplementary Fig. 2a–c ). The monoclonal cell population HSD SEAP32 (HSD SEAP clone 32) was the best-performing transgenic histamine-responsive cell line because it combined a very high SEAP induction factor (65-fold), superior absolute SEAP levels and an improved dynamic histamine-sensitivity range (1–10,000 nM) ( Fig. 1c ; Supplementary Fig. 2d ). A basic set of control experiments confirmed that, HEK-293 devoid of the HRH2 sensor module were insensitive to histamine ( Fig. 1d ), the metabolic integrity and viability of the cells as scored by constitutive SEAP expression were not impacted over the entire histamine concentration range ( Fig. 1d ) and histamine triggered an intracellular cAMP surge in double-transgenic HSD SEAP32 cells ( Fig. 1e ). In-depth characterization of the SEAP expression kinetics of HSD SEAP32 cells, cultivated for extended periods of time in medium containing specific histamine concentrations encompassing the physiological range, revealed extraordinarily low leakiness and a robust induction of the reporter gene over 3 days ( Fig. 1f ). Importantly, different induction pulse durations at physiological histamine concentrations in HSD SEAP32 cells revealed that high histamine levels rapidly activated transgene expression, whereas lower levels required a longer induction pulse period to reach significant SEAP secretion ( Fig. 1g ). Furthermore, cimetidine, an HRH2 antagonist, significantly reduced the reporter gene expression in HSD SEAP32 cells induced with 100 nM histamine, whereas cetirizine, a clinically licensed anti-allergy drug that acts as an HRH1 antagonist, did not impact the histamine-dependent SEAP expression profile of HSD SEAP32 cells ( Fig. 1h ) [23] . The allergy profiler is based on the crosslinking of membrane-bound high-affinity IgE receptors (FcεRI) via specific IgE–antigen complexes on immune effector cells, such as basophil granulocytes or mast cells, inducing a protein tyrosine kinase- and calcium (Ca 2+ )-dependent signal transduction cascade, which results in the release of a series of mediators, including histamine ( Fig. 2a ). We hypothesized that the exposure of human serum to HSD-engineered cells would mimic patient-specific in vivo allergic conditions and would lead to the corresponding production of the reporter gene in a manner that is precisely correlated to the basophil-derived histamine levels ( Fig. 2a ). As a preliminary step, we determined that a concentration of 12.5% (v/v) of human serum in cell culture medium provided the optimal dilution, as no effect on reporter gene expression was observed when exposing HSD SEAP32 to 100 nM histamine for 24 h ( Supplementary Fig. 3 ). Anti-IgE antibodies have been shown to efficiently crosslink IgE antibodies bound to FcεRI subsequently triggering histamine release from basophils ( Fig. 2a ) [24] . Therefore, we incubated increasing concentrations of a polyclonal anti-IgE antibody with heparinized human whole blood and exposed the resulting human serum for 24 h to HSD SEAP32 designer cells or to HEK-293 cells transiently transfected with control reporter plasmids (pcDNA3.1/pCK53) ( Fig. 2b ). We observed that increasing anti-IgE antibody concentrations induced basophil histamine release and, as a result, also induced a robust and gradual reporter gene expression response in the HSD SEAP32 cells, whereas no SEAP induction was observed when cells were incubated with the degranulation buffer alone (spontaneous release) ( Fig. 2b ). In contrast, no induction of SEAP activity was detected in transiently transfected control cells lacking the HRH2 sensor module, indicating that the reporter gene induction was specific to histamine and not to other potential mediator molecules present in human serum ( Fig. 2b ). Further, the HSD SEAP32 cell responses were dependent on the degranulation of effector cells: the inhibition of crucial protein tyrosine kinases in the intracellular signalling pathway of basophils by dasatinib, a multi-targeted tyrosine kinase inhibitor, abolished anti-IgE antibody-mediated reporter gene expression ( Fig. 2c ) [25] . As expected, the IgE-independent degranulation of basophils following N -formylmethionyl-leucyl-phenylalanine (fMLF) stimulation strongly induced SEAP expression of HSD SEAP32 cells as well ( Fig. 2d ) [26] . Finally, we profiled anti-IgE antibody- and fMLF-induced basophil degranulation of whole-blood samples taken from the same donor at different time points, which showed that HSD SEAP32 cells produced consistent values, considering that allergy profiles may slightly vary over time [17] . This validates the robustness and reliability of the HSD ( Supplementary Fig. 4 ). 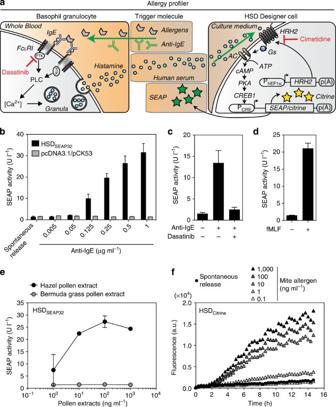Figure 2: Human basophil-derived histamine triggers reporter gene expression in HSD-engineered designer cells. (a) Illustration of the cell-dependent allergy profiler. Allergens added to the blood sample bind to IgE, which crosslink membrane-bound high-affinity IgE receptors (FcεRI) of basophil granulocytes. FcεRI activation induces a protein tyrosine kinase (PTK)- and phospholipase C (PLC)-dependent signal transduction cascade, resulting in an intracellular calcium (Ca2+) surge and a subsequent release of histamine. Histamine binds to HRH2 on the HSD designer cells and triggers dose-dependent reporter gene expression (seeFig. 1a). (b) Adjustable anti-IgE antibody-mediated basophil degranulation triggered SEAP secretion in HSDSEAP32cells, but not in pcDNA3.1/pCK53-co-transfected control cells lacking the HRH2 sensory module. (c) Inhibition of protein tyrosine kinases by dasatinib (1 μM) in basophils inhibited anti-IgE antibody-mediated degranulation (0.25 μg ml−1anti-IgE) and, therefore, HSDSEAP32-mediated reporter gene expression. (d) Detection of histamine derived from the IgE-independent fMLF-mediated induction of basophil degranulation (1 μM fMLF) by HSDSEAP32cells. (e) HSDSEAP32cells specifically converted hazel pollen-triggered histamine from an allergic donor to a reporter gene response, whereas Bermuda grass pollens repressed the designer cell responses. (f) Real-time detection of histamine derived from mite-induced basophil degranulation by HSDCitrine-engineered cells. The data represent the means±s.d. (n≥3 experiments). Figure 2: Human basophil-derived histamine triggers reporter gene expression in HSD-engineered designer cells. ( a ) Illustration of the cell-dependent allergy profiler. Allergens added to the blood sample bind to IgE, which crosslink membrane-bound high-affinity IgE receptors (FcεRI) of basophil granulocytes. FcεRI activation induces a protein tyrosine kinase (PTK)- and phospholipase C (PLC)-dependent signal transduction cascade, resulting in an intracellular calcium (Ca 2+ ) surge and a subsequent release of histamine. Histamine binds to HRH2 on the HSD designer cells and triggers dose-dependent reporter gene expression (see Fig. 1a ). ( b ) Adjustable anti-IgE antibody-mediated basophil degranulation triggered SEAP secretion in HSD SEAP32 cells, but not in pcDNA3.1/pCK53-co-transfected control cells lacking the HRH2 sensory module. ( c ) Inhibition of protein tyrosine kinases by dasatinib (1 μM) in basophils inhibited anti-IgE antibody-mediated degranulation (0.25 μg ml −1 anti-IgE) and, therefore, HSD SEAP32 -mediated reporter gene expression. ( d ) Detection of histamine derived from the IgE-independent fMLF-mediated induction of basophil degranulation (1 μM fMLF) by HSD SEAP32 cells. ( e ) HSD SEAP32 cells specifically converted hazel pollen-triggered histamine from an allergic donor to a reporter gene response, whereas Bermuda grass pollens repressed the designer cell responses. ( f ) Real-time detection of histamine derived from mite-induced basophil degranulation by HSD Citrine -engineered cells. The data represent the means±s.d. ( n ≥3 experiments). Full size image To examine whether HSD SEAP32 cells possess the ability to convert allergen-triggered basophil-derived histamine from human whole blood into a quantitative reporter gene expression response, we used blood from a donor with a clinical history of allergy against hazel pollen and exposed it to different concentrations of crude allergen extracts of hazel and Bermuda grass pollens. We found that the response of the allergy profiler directly correlated with the histamine levels derived from hazel pollen-mediated degranulated basophils, and that the signal was converted to an allergen-specific SEAP response profile ( Fig. 2e ). Importantly, HSD SEAP32 cells showed no activation when the diluted blood was amended with Bermuda grass pollen, thereby confirming the absence of an allergic reaction ( Fig. 2e ). Similarly, a donor with a known mite allergy was chosen to determine whether HSD Citrine -engineered cell populations could facilitate the real-time detection of histamine-induced gene expression derived from human basophils with an allergic response when exposed to different concentrations of a crude allergen extract of mites. Importantly, histamine from spontaneous release and the allergen at the lowest concentration showed the same fluorescence profile, whereas all of the other tested concentrations triggered a gradual cellular fluorescence response, which was detectable 3 h after histamine-containing human serum was added to the engineered cell population ( Fig. 2f ). Finally, we established a low-volume version of the allergy profiler, which was performed in 96-well plates, and applied it to whole-blood samples from four different human donors, including three allergic and one non-allergic subject. We expanded the allergen set to seven common allergens and profiled the potential allergic reactions using HSD SEAP32 cells. Importantly, our experimental design included relevant quality controls, such as spontaneously released histamine as a baseline control, anti-IgE antibody at three different concentrations and fMLF as a non-IgE-mediated positive control to provide information on donor-specific basophil sensitivity [27] , [28] . To acquire the maximum amount of information regarding potential allergic reactions, we used allergens at concentrations encompassing five orders of magnitude, that is, from 100 pg ml −1 to 1 μg ml −1 . The data were illustrated using a heat map, which provides a simple but detailed personalized allergy profile ( Fig. 3a ). In all allergy profiles, controls activated the designer cells as expected: spontaneous release produced baseline responses in HSD SEAP32 cells, whereas both anti-IgE antibody- and fMLF-mediated basophil degranulation triggered robust levels of reporter gene expression ( Fig. 3a ). Furthermore, the results of the allergy profiler revealed that two of three allergic donors exhibited a strong allergic reaction to three types of pollens, and one of them also showed a strong response to grass pollens. A specific allergy against mites was detected in one subject, whereas the non-allergic blood donor did not exhibit any allergen-dependent designer cell response ( Fig. 3a ). Most importantly, the scores of the allergy profiler correlated with the results of the skin prick test that is the current gold standard for allergy testing ( Fig. 3b ). We observed low intra-assay variability ( Supplementary Fig. 5 ) and high reproducibility of the allergy profile of donors B and C when profiling the same histamine release samples after two freeze–thaw cycles with another batch of HSD SEAP32 cells ( Supplementary Fig. 6 ). Also, HSD Citrine -engineered cells exposed to serum samples of donor B enabled real-time monitoring of Citrine production of the allergy profiler and provided allergy scores matching those achieved with HSD SEAP32 cells ( Fig. 4 ). 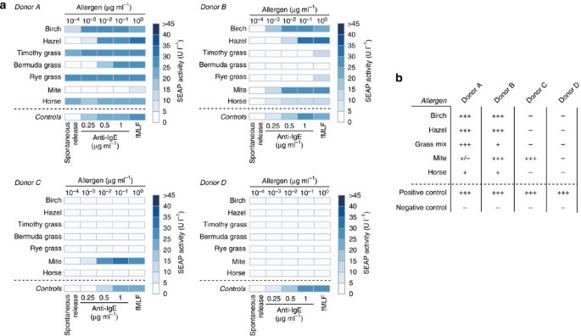Figure 3: Personalized allergy profiles of four human subjects. (a) Heat maps showing histamine-triggered HSDSEAP32cell responses to allergen-triggered basophil degranulation for four different donors. The allergen concentrations encompassed five orders of magnitude (1 μg ml−1–100 pg ml−1). The spontaneous release of histamine served as a negative control, and three different concentrations of anti-IgE antibody and 1 μM fMLF were used as positive controls. Each cell of the heat map shows the mean of two histamine release assays. (b) Skin prick test results. Tests were performed and evaluated by dermatologists at Swiss allergy centers according to standard protocols. All tests were validated in comparison with positive controls (10 mg ml−1histamine) and negative controls (diluent). Figure 3: Personalized allergy profiles of four human subjects. ( a ) Heat maps showing histamine-triggered HSD SEAP32 cell responses to allergen-triggered basophil degranulation for four different donors. The allergen concentrations encompassed five orders of magnitude (1 μg ml −1 –100 pg ml −1 ). The spontaneous release of histamine served as a negative control, and three different concentrations of anti-IgE antibody and 1 μM fMLF were used as positive controls. Each cell of the heat map shows the mean of two histamine release assays. ( b ) Skin prick test results. Tests were performed and evaluated by dermatologists at Swiss allergy centers according to standard protocols. All tests were validated in comparison with positive controls (10 mg ml −1 histamine) and negative controls (diluent). 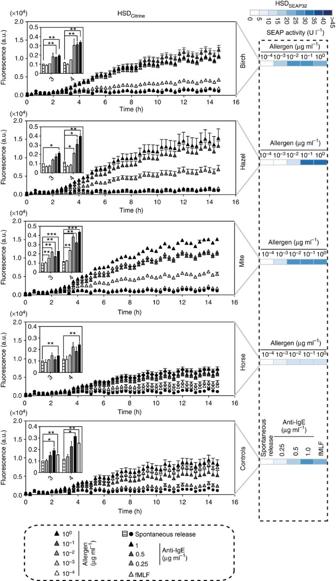Figure 4: Real-time monitoring of basophil-derived histamine in human serum. Histamine release assays were performed using blood of the allergic donor B including controls with buffer alone (spontaneous release), three different concentrations of anti-IgE antibody, an IgE-independent positive control (1 μM fMLF) as well as with five different concentrations of indicated allergens. HSDCitrine-engineered cell populations were exposed to human serum samples and the cellular fluorescence was monitored every 20 min using a microplate reader. Cells were cultured in a 5% CO2atmosphere at 37 °C. HSDSEAP32-mediated reporter gene expression profiles using the same serum samples are shown for comparison (see alsoFig. 3a). The insert shows bar graphs of cellular fluorescence of HSDCitrinecells at time points when differences between allergen-induced and spontaneous histamine release become statistically significant. Statistical analysis by a two-tailed Student’st-test (*P<0.05, **P<0.01 and ***P<0.001). Data represent means ±s.d of two histamine release assays. Full size image Figure 4: Real-time monitoring of basophil-derived histamine in human serum. Histamine release assays were performed using blood of the allergic donor B including controls with buffer alone (spontaneous release), three different concentrations of anti-IgE antibody, an IgE-independent positive control (1 μM fMLF) as well as with five different concentrations of indicated allergens. HSD Citrine -engineered cell populations were exposed to human serum samples and the cellular fluorescence was monitored every 20 min using a microplate reader. Cells were cultured in a 5% CO 2 atmosphere at 37 °C. HSD SEAP32 -mediated reporter gene expression profiles using the same serum samples are shown for comparison (see also Fig. 3a ). The insert shows bar graphs of cellular fluorescence of HSD Citrine cells at time points when differences between allergen-induced and spontaneous histamine release become statistically significant. Statistical analysis by a two-tailed Student’s t -test (* P <0.05, ** P <0.01 and *** P <0.001). Data represent means ±s.d of two histamine release assays. Full size image With the advent of synthetic biology there has been significant progress in the engineering of mammalian cells for biomedical applications [1] , [3] , [4] , [29] . Here, we describe the construction, characterization and validation of designer cells that sense the levels of the allergy mediator histamine in whole-blood samples and produce a corresponding cellular response that provides a robust and reliable diagnostic allergy profile. The allergy profiler represents a novel cell-based detection method for histamine originating from biological samples and combines extraordinary sensitivity (2–4 nM), a wide dynamic range (1–10,000 nM) and the flexibility to use different reporter genes with improved kinetics (rapid real-time detection of intracellular fluorescent proteins) or storage capacity (long-term storage of SEAP-containing supernatants). The allergy scores provided by the allergy profiler qualitatively correlate with the results of the skin prick test. However, since the allergy profiler scores histamine levels in an all- in vitro format without exposing the subject directly to potential allergens, such as the skin prick test, it could be used to diagnose allergies in infants and patients with skin disorder. Also, unlike the skin prick test, which semi-quantitatively scores the response to a single concentration of a specific allergen, the allergy profiler provides increased accuracy by recording the allergic response to an allergen concentration range of five orders of magnitude. Besides the skin prick test, there are a variety of diagnostic allergy tests that use antibody-based detection of basophil mediators. However, diagnostic antibodies are produced in classic biopharmaceutical production and downstream processing scenarios, which are expensive and prone to batch-to-batch variations. Most importantly, antibody-based detection of small molecules remains challenging and often requires modification of the target compound. Therefore, for most state-of-the-art diagnostic assays, histamine needs to be derivatized to achieve sensitivity in the clinical range, which is based on error-prone and time-consuming sample preparation procedures. In contrast, receptor-based detection of small-molecule compounds by designer cells takes advantage of the highly sensitive interaction of natural histamine with its receptor while producing the HSD in situ . Therefore, standardized designer cells provide a robust, reliable and highly sensitive one-step histamine-detection procedure. Capitalizing on its compatibility with a 96-well culture format, the allergy profiler is amenable to automated high-throughput liquid handling platforms to routinely provide highly detailed personalized allergy profiles for a larger population. Since HSD SEAP32 cells were also sensitive to clinically licensed HRH2 antagonist cimetidine and were able to monitor the inhibition of degranulation using the kinase inhibitor dasatinib, the allergy profiler may also be used as a cell-based screening assay for the discovery of anti-inflammatory and anti-allergic drugs. Cell-based assays have been shown to provide not only reliable drug–target interactions but also corresponding information on cytotoxicity and bioavailability [5] , [30] , [31] . Since the key factors of the pharmaceutical industry have declared personalized medicine—the interplay between diagnostics and therapeutic interventions—the treatment concept of the future diagnostics have come into the limelight as a powerful technology to detect and prevent high-prevalence medical conditions [32] . In the not-too-distant future, designer cells engineered with an array of human sensor components and programmed to interface with disease-effector molecules will provide novel standardized diagnostic opportunities for the detection, quantification and prevention of human diseases such as allergies, thereby paving the way for a new wave of synthetic biology-inspired ‘real-world’ applications [33] . Plasmid construction See Supplementary Table 1 . Cell culture Chinese hamster ovary cells (CHO-K1, ATCC: CCL-61) were cultivated in ChoMaster HTS (Cell Culture Technologies, Gravesano, Switzerland) supplemented with 5% (v/v) fetal calf serum (FCS; BioConcept, Allschwil, Switzerland; lot no. PE01026P) and a 1% (v/v) penicillin/streptomycin solution (Sigma-Aldrich, Munich, Germany). Human embryonic kidney cells (HEK-293, ATCC: CRL-11268), human cervical carcinoma cells (HeLa, ATCC: CCL-2) and baby hamster kidney cells (BHK-21, ATCC: CCL10) were cultured in Dulbecco’s modified Eagle’s medium (DMEM, Life Technologies, Carlsbad, CA, USA) supplemented with 10% FCS and a 1% penicillin/streptomycin solution. All of the cells were cultured at 37 °C in a humidified atmosphere containing 5% CO 2 . Cell numbers and viability were quantified using an electric field multi-channel cell-counting device (CASY Cell Counter and Analyzer Model TT; Roche Diagnostics GmbH, Basel, Switzerland). For transfection, a solution containing 0.15–0.25 μg of plasmid DNA (SEAP output: 125 ng of pCK120/25 ng of pCK5; Citrine output: 50 ng of pCK120/200 ng of pDA134) and 2 μl PEI (1 mg ml −1 ) was incubated in 0.05–0.1 ml of FCS-free DMEM for 30 min at 22 °C before being added dropwise to 2.5 × 10 4 –5 × 10 4 cells seeded per well of a 96-well or 48-well plate 16 h before transfection. Unless stated otherwise, the transfection medium was replaced by standard cultivation medium after 7 h. After an additional 16 h, the cells were induced by adding standard cultivation medium supplemented with the indicated amounts of chemical inducers, including histamine dihydrochloride (cat. no. H7250, Sigma), cetirizine (cat. no. C3618, Sigma) or cimetidine (cat. no. C4522, Sigma). The transgene expression was then profiled after 24 h. Design of transgenic cell lines To develop the transgenic cell lines, HEK-293 cells were co-transfected with pCK120 (1.5 μg)/pCK53 (1 μg) in one well of a six-well plate; after 7 h, the medium was changed to normal DMEM. After 48 h, the cells were transferred to a 10-cm dish, and a stable polyclonal cell population (HSD SEAP-polyclonal ) was selected for 3 weeks in DMEM supplemented with 20 μg ml −1 blasticidin (cat. no. ANT-BL-1, LabForce AG, Switzerland). Subsequently, monoclonal cell populations were selected by limiting dilution and were grown for an additional 2 weeks in blasticidin-containing DMEM. Individual clones were screened for histamine-responsive SEAP expression, and HSD SEAP32 was chosen for further experiments. Stable cell populations between passages 4–10 were used for subsequent experiments. Analytical assays cAMP. Intracellular cAMP levels were quantified using the Cyclic AMP XP Assay Kit (cat. no. 4339, Life Technologies). In brief, 1 × 10 5 cells were pretreated for 30 min with 0.5 mM 3-isobutyl-1-methylxanthine (IBMX, cat. no. I5879, Sigma) in FCS-free DMEM. The cells were incubated for an additional 30 min in FCS-free DMEM supplemented with the indicated concentrations of histamine hydrochloride before the intracellular cAMP levels were determined in cell lysates according to the manufacturer’s protocol. SEAP . The production of human placental-secreted alkaline phosphatase was quantified in cell culture supernatants as previously described [34] . Cellular fluorescence . The cellular fluorescence of cell populations cultured in a 5% CO 2 atmosphere at 37 °C in 96-well plates was profiled every 20 min using a monochromatic Tecan Infinite M200 PRO plate reader (Tecan Group Ltd, Männedorf, Switzerland) at an excitation and emission of 491/9 nm and 530/20 nm, respectively. The autofluorescence of mock-transfected cells was subtracted from the fluorescence of cells containing allergy profiler components. Allergens Crude allergen extracts, including Betula alba pollen (white birch, cat. no. P6770, Sigma), Corylis avellana pollen (hazel, cat. no. 0127, Allergon AB, Ängelholm, Sweden), Cynodon dactylon pollen (Bermuda grass, cat. no. 0421, Allergon AB), Phleum pratense (timothy grass, cat. no. 0113, Allergon AB), Lolium perenne pollen (perennial rye grass, cat. no. 0214, Allergon AB), Dermatophagoides pteronyssinus allergen (house dust mite, cat. no. 4965, Allergon AB) and Equus caballus allergen (horse dander, cat. no. 2046, Allergon AB) were dissolved in degranulation buffer (25 mM piperazine- N , N ′-bis(2-ethanesulfonic acid) (cat. no. 80635, Sigma), 110 mM sodium chloride (cat. no. S7653, Sigma), 5 mM potassium chloride (cat. no. P9541, Sigma) and 0.01% (v/v) thimerosal (cat. no. T8784, Sigma); pH 7.4), and each mixture was stirred at 300 r.p.m. at 4 °C for 16 h. Subsequently, each allergen mixture was centrifuged, the supernatant was filter-sterilized and the total protein concentration was measured using the Bradford assay. The allergen solutions were stored at −20 °C at a concentration of 1 mg ml −1 . Histamine release from human basophils Peripheral blood was drawn from healthy donors after obtaining written consent. The study was approved by the Ethics Committee of the ETH Zurich (no. EK 2012-N-42). A 100-μl aliquot of heparinized whole blood was mixed with 100 μl of degranulation buffer supplemented with the indicated concentrations of allergen, anti-IgE antibody (goat anti-human IgE antibody, cat. no. AP175, lot no. 2101963; Merck Millipore AG, Billerica, MA, USA), or N -formylmethionyl-leucyl-phenylalanine (fMLF, cat. no. 47729, Sigma) in one well of a U-shaped bottom 96-well plate (cat. no. 650185, Greiner Bio One, Austria). The histamine release assay was performed in an incubator at 37 °C in a humidified 5% CO 2 -containing atmosphere for 30 min. Thereafter, the cells were centrifuged for 10 min at 700 g at 4 °C. The resulting serum was either directly used for subsequent assays or was stored at −20 °C. Cell-based allergy test SEAP output. Unless stated otherwise, 5 × 10 4 HSD SEAP32 cells were seeded into each well of a 96-well plate containing 105 μl of standard cultivation medium. After 12 h, 15 μl of human serum derived from histamine release assays was added, and the cells were incubated for an additional 24 h. The supernatant was collected and either directly used for analytical assays or stored at −20 °C until SEAP quantification. Citrine output. A total of 5 × 10 4 HEK-293 cells were seeded into each well of a 96-well plate with a transparent bottom (cat. no. 655090, Greiner Bio One) 16 h before the co-transfection of 50 ng of pCK120 and 200 ng of pDA134, resulting in HSD Citrine -engineered cells. After 7 h, the transfection medium was replaced with 105 μl of standard cultivation medium, and 15 μl of human serum was added to the cells. The cells were cultivated in a microplate reader (Infinite M200 PRO plate reader, Tecan Group Ltd) in a 5% CO 2 atmosphere at 37 °C for 16 h, and the cellular fluorescence was quantified in real time as described above. How to cite this article: Ausländer, D. et al . A designer cell-based histamine-specific human allergy profiler. Nat. Commun. 5:4408 doi: 10.1038/ncomms5408 (2014).